Interlaced crystals having a perfect Bravais lattice and complex chemical order revealed by real-space crystallography The search for optimal thermoelectric materials aims for structures in which the crystalline order is disrupted to lower the thermal conductivity without degradation of the electron conductivity. Here we report the synthesis and characterisation of ternary nanoparticles (two cations and one anion) that exhibit a new form of crystalline order: an uninterrupted, perfect, global Bravais lattice, in which the two cations exhibit a wide array of distinct ordering patterns within the cation sublattice, forming interlaced domains and phases. Partitioning into domains and phases is not unique; the corresponding boundaries have no structural defects or strain and entail no energy cost. We call this form of crystalline order ‘interlaced crystals’ and present the example of hexagonal CuInS 2 . Interlacing is possible in multi-cation tetrahedrally bonded compound with an average of two electrons per bond. Interlacing has minimal effect on electronic properties, but should strongly reduce phonon transport, making interlaced crystals attractive for thermoelectric applications. We discovered the novel crystalline structures during an investigation of CuInS 2 semiconductor nanoparticles that are actively studied for solar energy harvesting and other applications [1] , [2] , [3] , [4] , [5] . They often have the chalcopyrite structure of bulk CuInS 2 , that is, a zinc-blende structure in which Cu and In share the cation sublattice [1] , [2] . Some methods of synthesis, however, yield nanoparticles that have a hexagonal structure, the wurtzite analogue of chalcopyrite [1] , [3] , [4] , [5] . These hexagonal CuInS 2 nanoparticles are believed to be single crystals with an ordered sulfur sublattice, but it has not been established whether the Cu and In atoms are randomly distributed or ordered (it should be noted that the words lattice and structure are used differently by the physics and crystallography community; we use the physics terminology where lattice is a mathematical abstraction). From theory, ordered cations are favoured over random distributions of cations according to the Grimm–Sommerfeld (GS) or valence-octet rule [6] , which has been confirmed by density functional theory (DFT) calculations for bulk cubic I-III-VI 2 [7] , [8] and related quaternary materials [9] . In cubic CuInS 2 thin films, X-ray diffraction (XRD) and transmission electron microscopy (TEM) [10] have established the coexistence of two ordered phases: chalcopyrite, which is the ground state, and a CuAu-like phase, which, according to theory [8] , is only slightly higher in energy. For nanoparticles, however, reciprocal-space X-ray crystallographic techniques yield patterns with broad, weak peaks. Thus, any small peaks and subtle changes in the pattern that would be diagnostic of the presence of one or several ordered phases are not discernible. Instead, only the average lattice (hexagonal in this case) is determined and the question of cation ordering in the wurtzite phase remains unanswered. Although the octet rule, which is backed by DFT calculations, enshrines the notion that ordered cations are energetically preferred over a random distribution, it does not specify if there is a preferred ordering or set of orderings or any potential distribution. The aim of the present paper is to present the experimental evidence for the manifestation of interlaced crystals and a theoretical rational for their existence. Here we use real-space crystallography in the form of Z-contrast imaging on an aberration-corrected scanning TEM (STEM), to directly distinguish the In and Cu atoms in the nanoparticles. We also employ DFT to determine an entire family of ordered hexagonal CuInS 2 phases (polytypes) that are essentially degenerate in energy and are favoured over phases with disordered cations in accord with the GS rule, as is the case for cubic CuInSe 2 (ref. 7 ). The two approaches independently yield the same result: the Cu and In cations are not randomly distributed in the cation sublattice of a wurtzite crystal structure. Instead the abstract cation sublattice retains its perfect structure while the two cation species exhibit a range of ordered structures. The key experimental finding is that the Z-contrast images show a continuum of interlaced phases and domains that can be demarcated in a variety of ways as illustrated in Fig. 1 , with an uninterrupted, perfect Bravais lattice. At the same time, the calculations found that phase and domain boundaries are defect- and strain-free and cost no energy, and confirm that the global Bravais lattice remains intact. As a further evidence, strain analysis of the Z-contrast images reveals that there is no measurable strain. We will further demonstrate that the partitioning into domains and phases is not unique and that domain boundaries are twins by either rotational or reflection symmetry (see Supplementary Information ), while phase boundaries have no twinning symmetry operation. It is the combination of a perfect, uninterrupted global Bravais lattice and the nonuniqueness of partitioning, with strain-free, defect-free domain and phase boundaries that characterises what we call ‘interlaced crystals’. Such crystallographic features are likely to exist in many similar compounds. 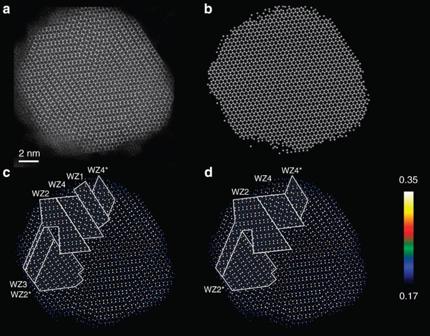Figure 1: Direct imaging of cation ordering in an interlaced CuInS2nanoparticle. (a) Unprocessed Z-contrast STEM annular dark field (ADF) image of a CuInS2nanoparticle. The image is taken along thecaxis of the wurtzite lattice, which is also the vertical axis of the pancake-shaped nanocrystal. (b) Simulated image based on the atomic positions extracted froma, with the same intensity at all atomic sites. (c,d) Different ways to partition the nanoparticle, demonstrating the interlacing nature of the cation ordering. The partitioning is done on the colourized low by-pass filtered ADF image to highlight the difference between Cu and In columns. The colour scale bar is shown ind. The dark level of the images is set to 0.17 and the maximum level is set to 0.35 for contrast enhancement, so that columns containing the heavier In cations display as yellow dots while columns containing the lighter Cu cations display as blue dots. (SeeSupplementary Fig. 4c,dfor more details.) The notion WZ2 and WZ4 refer to phases of CuInS2with different ways of cation ordering. The notation WZ2/WZ2* (and WZ4/WZ4*) is used to label different cation-ordering domains of the same phase but with different orientations. Over two hundred high-resolution images were taken from three batches of nanoparticle samples, and the interlaced crystal structure was consistently observed. Figure 1: Direct imaging of cation ordering in an interlaced CuInS 2 nanoparticle. ( a ) Unprocessed Z-contrast STEM annular dark field (ADF) image of a CuInS 2 nanoparticle. The image is taken along the c axis of the wurtzite lattice, which is also the vertical axis of the pancake-shaped nanocrystal. ( b ) Simulated image based on the atomic positions extracted from a , with the same intensity at all atomic sites. ( c , d ) Different ways to partition the nanoparticle, demonstrating the interlacing nature of the cation ordering. The partitioning is done on the colourized low by-pass filtered ADF image to highlight the difference between Cu and In columns. The colour scale bar is shown in d . The dark level of the images is set to 0.17 and the maximum level is set to 0.35 for contrast enhancement, so that columns containing the heavier In cations display as yellow dots while columns containing the lighter Cu cations display as blue dots. (See Supplementary Fig. 4c,d for more details.) The notion WZ2 and WZ4 refer to phases of CuInS 2 with different ways of cation ordering. The notation WZ2/WZ2* (and WZ4/WZ4*) is used to label different cation-ordering domains of the same phase but with different orientations. Over two hundred high-resolution images were taken from three batches of nanoparticle samples, and the interlaced crystal structure was consistently observed. Full size image Nanoparticle characterisation Nanoparticles of CuInS 2 were synthesized by a solution-phase colloidal synthesis at 245 °C [11] . Characterisation by TEM, XRD and UV–vis absorption spectrum analysis were performed. TEM shows that the nanoparticles have a pancake shape, with a diameter of 18±2 nm and thickness of 8±2 nm ( Supplementary Fig. 1 ). Powder XRD ( Fig. 2a ) verified that the structure is hexagonal, as it would be in a binary compound with the wurtzite structure. Scherrer broadening calculations of the strong (100)-like reflection at 26.8° yields a crystallite size of 20 nm ( Supplementary Fig. 2 and Supplementary Note 1 ), which is consistent with the TEM analysis. The XRD provides supporting evidence that there is an uninterrupted global Bravais lattice in the interlaced crystals, as the 20-nm size calculated from Scherrer broadening on wurtzite reflections is far larger than the 3–5-nm lateral size of cation-ordered domains observed in the STEM image ( Fig. 1a ). 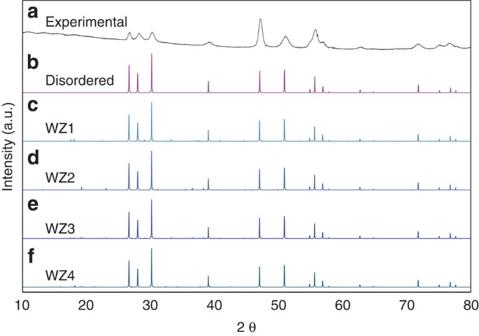Figure 2: Experimental and simulated XRD patterns. (a) XRD patterns of CuInS2nanoparticles, (b) simulated pattern for a hexagonal wurtzite structure with disordered cation sublattice and (c–f) simulated patterns for the four different ordered structures (seeFig. 3and Methods). Figure 2: Experimental and simulated XRD patterns. ( a ) XRD patterns of CuInS 2 nanoparticles, ( b ) simulated pattern for a hexagonal wurtzite structure with disordered cation sublattice and ( c – f ) simulated patterns for the four different ordered structures (see Fig. 3 and Methods). Full size image While the wurtzite reflections are clearly observed in the XRD pattern of nanoparticles, the reflections due to cation ordering are too low in intensity to be discerned. This is due to the combined effect of several factors: (1) the different ordered phases do not necessarily generate superlattice reflections at the same 2 θ ( Fig. 2 ), whereby the presence of multiple cation-ordered phases reduces the signal from each phase proportionally (in addition to the WZ1–WZ4 structures shown in Fig. 3 , other cation-ordered phases with similar band gaps are possible and would also weaken the superlattice reflections); (2) the natural intensities of these reflections are intrinsically low, as can be seen from Fig. 2c–f ; (3) Scherrer broadening is greater for the cation-ordered reflections than for the overarching wurtzite reflections ( Supplementary Note 1 ). 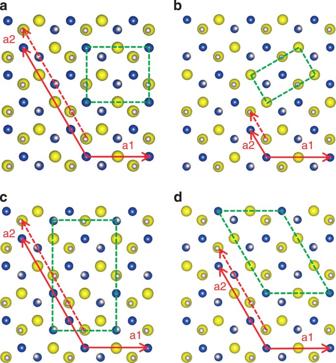Figure 3: Projection view of the four structures along the [001] direction with ordered cation sublattices. (a) WZ1, (b) WZ2, (c) WZ3 and (d) WZ4. Cu atoms are in blue, In atoms are in yellow and S atoms are in grey. The repeating Cu1–In1and Cux–Inyunits along the direction of the lattice vectors in the wurtzite structure are shown by red arrows. The ‘conjugated’ Inx–Cuyunits are shown as the dotted red arrows. The primitive unit cells are shown by green dashed lines. Figure 3: Projection view of the four structures along the [001] direction with ordered cation sublattices. ( a ) WZ1, ( b ) WZ2, ( c ) WZ3 and ( d ) WZ4. Cu atoms are in blue, In atoms are in yellow and S atoms are in grey. The repeating Cu 1 –In 1 and Cu x –In y units along the direction of the lattice vectors in the wurtzite structure are shown by red arrows. The ‘conjugated’ In x –Cu y units are shown as the dotted red arrows. The primitive unit cells are shown by green dashed lines. Full size image Indirect information about cation ordering is provided by the UV–vis absorption spectrum, which shows that the nanoparticles have a band gap of 1.55 eV ( Supplementary Fig. 3 ), close to that of the chalcopyrite CuInS 2 (1.54 eV) [12] . Indeed, DFT calculations find that a disordered cation sublattice results in a much smaller band gap than that of chalcopyrite CuInS 2 ( Supplementary Table 1 ). Real-space crystallography Figure 1a shows an unprocessed STEM Z-contrast image from the pancake-shaped CuInS 2 nanocrystals, taken along the c axis of the wurtzite lattice. Figure 1b shows a simulated image based on the atomic positions extracted from the image in Fig. 1a , assuming there is only one type of cation. It is clear from this image that the abstract cation sublattice of the structure is a perfect hexagonal Bravais lattice without any structural interfaces, such as stacking faults, twins or grain boundaries. As we will now demonstrate, however, the cations form several different ordered structures within the cation sublattice, creating interlaced domains that can be demarcated by domain boundaries, but the partitioning is not unique. The perfect Bravais anion and cation sublattices, and interlaced domains are the key features of what we call ‘interlaced crystals’. The colourized version of the STEM Z-contrast image ( Fig. 1c,d ) shows clearly that there are distinct Cu and In columns (blue and yellow, respectively), which means that the majority of Cu and In atoms do not occupy random sites in the cation lattice, as that would result in a roughly uniform intensity in all atomic columns throughout the nanoparticle. The Cu and In columns form a complex pattern that can be decomposed into a set of fundamental cation-ordered phases (WZ1–WZ4) shown in Fig. 3 and domains (as further confirmed by atomic-resolution elemental mapping shown in Supplementary Fig. 5 ). The coexistence of various cation-ordered phases is also confirmed by secondary spots in the simulated electron diffraction pattern ( Supplementary Fig. 6 ) and Fourier transform of the STEM image ( Supplementary Fig. 4b ). In addition to the chemical ordering, strain analysis of the Z-contrast images reveals that there is no measurable strain ( Supplementary Fig. 7 ). DFT calculations The peculiar structure of the interlaced crystals described in this paper originates from the bonding requirements in tetrahedrally coordinated I-III-VI 2 compounds such as CuInS 2 . To have an average of four electrons associated with each atom, which is optimal for tetrahedral bonds, the group-VI atom (S) must have two group I (Cu) neighbours and two group III (In) neighbours according to the GS or valence-octet rule [9] . In contrast, in isovalent ternary compounds like AlGaAs, the GS rule is always satisfied regardless of the distribution of cations. In these alloys, a disordered cation sublattice is favoured by entropy, as long as the size mismatch between the cations is not large [13] . For cubic CuInS 2 , the GS rule is satisfied in two known cubic structures: one is the chalcopyrite structure that is the ground state for CuInS 2 ; the other is the CuAu-like ordered structure, which is slightly higher in energy [8] and has been observed in thin films [10] . Wei et al. [7] identified a family of cubic polytypes for the similar CuInSe 2 whose energies are only slightly higher than that of the chalcopyrite ground state. We found that for the wurtzite-like hexagonal CuInS 2 , the GS rule results in a family of structures, including the four structures that are depicted in detail in Fig. 3 and were independently predicted by DFT calculations. The first two structures, which we call WZ1 and WZ2, are constructed by hexagonal analogies to the chalcopyrite and CuAu-like structures, respectively. The third structure, WZ3, was obtained by running a reverse Monte Carlo simulation [14] , which ensured that S atom has exactly 50% probability of finding Cu atom as its nearest neighbour. The common feature of structures WZ1, WZ2 and WZ3 is that their lattices are constructed by repeating a Cu 1 –In 1 unit in one direction and a Cu x –In y unit in another direction (with a ‘conjugated’ In x –Cu y arrangement a half-cell below). Therefore, there exists a family of an infinite number of orderings, characterised by non-negative integers x and y , that satisfies the GS/valence-octet rule. For the WZ1 structure, x=y=2. For the WZ2 structure, x=∞ and y=0. In the case of the WZ3 structure, x=3 and y=1. The next simplest member of the family is x=2 and y=1, which we label as WZ4. (For the structure data, see Supplementary Note 2 ). DFT total-energy calculations show that these structures are very close in energy (enthalpy), with WZ1 being slightly lower by <4 meV per CuInS 2 unit. As in the case of the cubic CuInSe 2 polytypes [7] , all four structures have significantly lower energy than structures with disordered cation sublattices ( Supplementary Table 2 ), where each unit of deviation from the GS rule (one Cu-S/In-S bond pair) costs 0.3~0.4 eV of energy. It is possible to interpret some of the structures as derivatives of others. For example, the WZ3 structure can be viewed as a derivative of WZ2 with twinning domains while WZ4 can be viewed as a derivative of WZ2 with slips. However, they are better described as distinct, ordered structures, because the derivative descriptions imply structural defects and do not fully capture the translational symmetries. One can extend the family of WZ n structures. While the repetition of a Cu 1 –In 1 unit in one direction is always required, the repetition of a Cu x –In y unit in the second direction is not necessary. We found that any combination of Cu and In, Cu x1 –In y1 –Cu x2 –In y2 –…, can result in a structure in which every S has two Cu and two In neighbours if there is a conjugated In x1 –Cu y1 –In x2 –Cu y2 –… arrangement a half-cell below. This feature makes the arrangement of Cu and In columns very flexible, allowing the coexistence of various phases of cation ordering and different orientations of cation-ordering domains, as observed experimentally in the nanoparticles. The calculated energies of domain and phase boundaries are essentially zero ( Supplementary Table 3 ). One important consequence of the existence of a perfect global Bravais lattice is that the structure can be partitioned into domains and phases in a nonunique way as illustrated in Fig. 1c,d , where we show two different ways of partitioning part of the image into the fundamental ordered structures. In Fig. 1c , we divide the structure into six parts, two WZ2 domains, two WZ4 domains, a WZ1 phase and a WZ3 phase. In Fig. 1d , we divide the same particle into only four parts: two WZ2 and two WZ4 domains. The nonuniqueness of partitioning occurs because the different phases are not stacked along the z -direction ( c axis), which would yield a superlattice of polytypes. In such stacking, the phase boundaries would not obey the GS rule. In these nanoparticles, however, different phases are primarily juxtaposed as columns in the xy plane, that is, the nanoparticles can be described as textured [15] and the GS rule is obeyed without interruption. The 60° boundary between two WZ2 domains is equivalent to a piece of WZ3 structure, and the boundary between two WZ4 domains is equivalent to a piece of WZ1 structure. A boundary between two domains of the same phase yielding a different stable phase is a feature that has not been observed in other material systems. The interlaced nature of the crystal structure not only shows up at domain boundaries, but also at phase boundaries. The boundary between WZ2 and WZ4 phases is assigned differently in Fig. 1c,d . 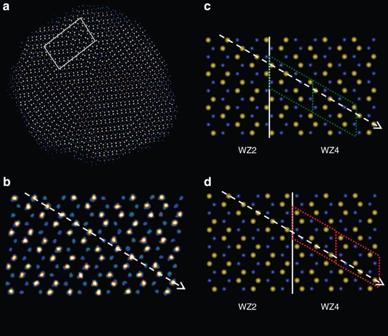Figure 4: Nonunique partition of ordered domains in the interlaced crystal. (a) Z-contrast STEM image of a nanoparticle, with the area of interest marked. (b) Enlarged view of the area of interest. (c,d) Two different ways to partition the area into WZ2 and WZ4 structures, demonstrating the interlaced lattice. The solid white line shows the position of the phase boundary. The dashed white arrow marks the –In5–Cu–In2–Cu–In2– arrangement of Cu and In atoms discussed in the text. Each green and red box shows a unit cell of the repeating WZ4 structure on the right. To illustrate the phenomenon more clearly, we zoom in to the area around the boundary ( Fig 4a,b ). An –In 5 –Cu–In 2 –Cu–In 2 – arrangement is marked with a dotted white arrow that crosses the two phases. The position of the phase boundary could be assigned at multiple locations with the extremes illustrated in Fig. 4c,d . Therefore, the middle section belongs to both the WZ2 and the WZ4 structures, making the two phases interlaced. We note that, in addition to the I-III-VI 2 and related materials, there have been other cases where two cations share the same sublattice and cation ordering occurs in domains, for example, in perovskite-structure transition-metal oxides [16] , [17] . However, in these systems the local changes in stoichiometry increase the Coulombic repulsions between cations, perturb the anion sublattice and raise the free energy [16] . Such distortions and associated energy costs are typical in all cases of structural boundaries, such as grain boundaries, twin boundaries and stacking faults. Even coherent twin boundaries were recently reported to entail distortions and energy costs [18] . In contrast, in what we call interlaced crystals, the local bonding at both domain and phase boundaries is the same as in the bulk crystal, without any distortions, disruptions or energy cost. Figure 4: Nonunique partition of ordered domains in the interlaced crystal. ( a ) Z-contrast STEM image of a nanoparticle, with the area of interest marked. ( b ) Enlarged view of the area of interest. ( c , d ) Two different ways to partition the area into WZ2 and WZ4 structures, demonstrating the interlaced lattice. The solid white line shows the position of the phase boundary. The dashed white arrow marks the –In 5 –Cu–In 2 –Cu–In 2 – arrangement of Cu and In atoms discussed in the text. Each green and red box shows a unit cell of the repeating WZ4 structure on the right. Full size image Although the domain boundaries in CuInS 2 can be identified as a form of twinning [19] , [20] , they exhibit an unbroken global Bravais lattice, which is not a feature of any known twin boundaries ( Supplementary Fig. 8 and Supplementary Note 3 ). The phase boundaries in CuInS 2 , on the other hand, are definitely not twins as they lack a twinning symmetry operation. All boundaries are defined strictly through the ordering of the cations in the otherwise perfect Bravais lattice, which underlies the nonuniqueness of the partitioning. It is for these reasons that the order observed in CuInS 2 nanoparticles is a prototype of a new form of crystalline order. Although the size and shape of the nanoparticles have facilitated this discovery, (the small thickness allows for clear Z-contrast between the In and Cu columns, and the pancake-shaped particles lie flat so that the c axis is conveniently observed with Cu and In columns easily distinguished), each nanoparticle contains ~50,000 atoms, and thus surface energy contributions are likely low. Therefore, the observed crystalline behaviour is bulk-like and not intrinsic to nanoparticles. We expect that interlaced crystals should exist in thin films and bulk materials as well. If the size of ordering phase and domain in these materials is ~5 nm as observed in the present study, XRD analysis is likely to be insufficient to identify the cation-ordered phases. The very weak reflections ( Fig. 2c–f ) due to cation ordering will have a line broadening of 1.8° ( Supplementary Note 1 ), which makes them difficult to be observed. In addition to hexagonal CuInS 2 and other I-III-VI 2 compounds, interlacing is likely to occur in cubic versions of these materials, in II-IV-V 2 compounds such as ZnGeAs 2 or ZnGeP 2 and in I 2 -II-IV-VI 4 quaternaries. Such materials have been synthesized and have been found to exhibit ordering in the cation sublattice in accord with the GS rule and DFT calculations [21] , [22] . In addition, anti-phase boundaries in ZnGeAs 2 were observed by TEM 25 years ago [21] , and could be described by the interlacing phenomena. In all cases modern Z-contrast imaging could verify the presence of interlaced crystal ordering. Interlaced crystals are expected to have contrasting electronic and phonon mobilities due to the nonunique assignment of phase boundaries and domain structure. Unlike grain boundaries in polycrystalline materials, the local bonding at domain and phase boundaries in an interlaced crystal is the same as in the bulk, with no mismatched or distorted bonds. Therefore, the domain and phase boundaries of interlaced crystals should have minimal effect on electron transport. In contrast, phonon transport should be reduced significantly. Phonon scattering happens at not only phase boundaries because of their different phonon spectra, but also at domain boundaries, as it is impossible to conserve both the phonon wavevector and vibrational eigenvector due to the different orientation of the domains. The existence of such a phonon scattering mechanism at domain boundaries has been demonstrated at ferroelectric domain walls [23] . As a result, interlaced crystals should have high electron conductivities but low phonon conductivities, which make them ideal for thermoelectric applications. Recently, a high figure of merit of 1.4 was reported for bulk chalcopyrite CuGaTe 2 (ref. 24 ). Interlaced crystalline order is possible in such materials and is the likely source of the high thermoelectric performance. Future efforts to control crystallisation in the mixed cation copper chalcogenides and encourage a high density of interlaced crystal domains, should yield new thermoelectric materials with even higher figures of merit. Nanocrystal synthesis CuCl (99.99%, STREM), InCl 3 (99.99%, Alfa Aesar), thiourea (ACS reagent ≧ reagen Sigma-Aldrich), oleylamine (technical grade 70% Aldrich) were used as received. The CuInS 2 nanoparticles were synthesized following the procedure reported in ref. 11 , CuCl (0.5 mmol), InCl 3 (0.5 mmol), thiourea (1.0 mmol) and oleylamine (10.0 ml) were loaded on a 25-ml 3-neck flask containing a stir bar. The flask was equipped with a condenser connected to a vacuum/purging adaptor, as well as a thermocouple and two septa. The mixture was placed under vacuum at 60 °C for 30 min, then heated to 245 °C under nitrogen and held at this temperature for 1 h after which the heating mantle was removed. After cooling to room temperature, the particles were precipitated with ethanol followed by centrifugation and removal of the supernatant. Three cycles were performed of suspension in hexanes:oleylamine (20:1, by volume) followed by precipitation by excess ethanol, centrifugation and removal of the supernatant. Finally, the nanocrystals were stored in hexanes:oleylamine. Low-resolution TEM, XRD and UV–vis absorption spectrum Low-resolution TEM was carried out on a Phillips CM20 operating at 200 kV. The powder XRD pattern was collected over 43 h on an Inel powder diffractometer equipped with a curved position-sensitive detector (CPS 120) and a Cu Kα 1 radiation source operated at 40 kV and 20 mA. The software Powder Cell was employed for the simulation of the diffraction patterns from DFT results of ordered structures. To fit the positions of major peaks to that of experiment, the DFT lattice constants are adjusted (the a and c parameters of the underlying wurtzite lattice are scaled to 3.86 and 6.37 Å, respectively). UV–vis absorption spectrum was collected on a Jasco V-670 spectrophotometer. Reverse Monte Carlo The WZ3 structure and two structures with disordered cation sublattices were generated using a reverse Monte Carlo algorithm in a 128-atom supercell, which corresponds to a 4 × 4 × 2 supercell of the wurzite structure. The cost function in reverse Monte Carlo simulation is , where n I is the number of group I atoms and N is coordination number (which equals four in this material). The starting state of the simulation is a random distribution of 50% of Cu and 50% of In atoms in the cation site. For generating the WZ3 structure, the minimisation of cost function stops when it equals zero, which corresponds to every S atom in the simulation cell having exactly 50% probability of finding Cu as nearest neighbour (two Cu atoms out of four nearest neighbours). For generating the two structures with disordered cation sublattices, the minimisation stopped when the cost function is close to zero, therefore ensuring that each group-VI atom had close to 50% probability of finding a group I atom as its nearest neighbour, while retaining some randomness in the cation sublattice, which is characterised by an increased number of same-type neighbour pairs in the cation sublattice as compared with the ordered configurations. DFT calculations The band gaps are obtained from hybrid density functional theory calculations using the PBE0 version of the exchange-correlation functional [25] . The cohesive energies are obtained using DFT calculations with the PBE version of the exchange-correlation functional [26] . We employed PAW potentials [27] and plane-wave basis as implemented in the VASP code [28] . We used 400 eV for the plane-wave cutoff. The geometrical optimizations are converged to 10 −4 eV for the energy difference between two ionic steps. The energies of domain and phase boundaries are obtained using DFT calculations with the PBE functional. The calculations are done in 12 × 2 × 1 supercell of the wurzite structure with 96 atoms, which contains a pair of the boundaries. The energies of the boundaries are calculated by subtracting the total energies of the respective bulk phases from the total energy of the boundary model. High-resolution electron microscopy characterisation The high-resolution STEM imaging and electron energy loss spectroscopy analysis were performed with an aberration-corrected Nion UltraSTEM-100 operated at 100 kV accelerating voltage. The convergence semi-angle for the incident probe was 31 mrad and the annular dark field images were acquired with a collection semi-angle range of about 86–200 mrad. EEL spectra were collected using a Gatan Enfina spectrometer with an EELS collection semi-angle of 48 mrad. Energy dispersion of 1 eV per channel was used for the elemental mapping. The atomic position in the annular dark field image was extracted using the standard ‘Fine Maxima’ in ImageJ. Electron diffraction simulation was performed using SingleCrystal plug-in within CrystalMaker ( http://www.crystalmaker.com/ ). Strain field analysis was performed using a GPA analysis plug-in ( http://www.christophtkoch.com/strain/index.html ). How to cite this article: Shen, X. et al. Interlaced crystals having a perfect Bravais lattice and complex chemical order revealed by real-space crystallography. Nat. Commun. 5:5431 doi: 10.1038/ncomms6431 (2014).